Electric-field control of domain wall motion in perpendicularly magnetized materials Domain wall motion in materials exhibiting perpendicular magnetic anisotropy has been the subject of intensive research because of its large potential for future spintronic devices. Recently, it has been shown that perpendicular anisotropy of thin films can be influenced by electric fields. Voltage-controlled magnetic switching has already been realized, which is envisioned to lead to low-power logic and memory devices. Here we demonstrate a radically new application of this effect, namely control of domain wall motion by electric fields. We show that an applied voltage perpendicular to a Co or CoB wire can significantly increase or decrease domain wall velocities. Velocity modification over an order of magnitude is demonstrated (from 0.4 to 4 μm s −1 ), providing a first step towards electrical control of domain wall devices. This opens up possibilities of real-time and local control of domain wall motion by electric fields at extremely low power cost. Domain wall (DW) motion in materials exhibiting perpendicular magnetic anisotropy (PMA) is a highly interesting phenomenon for future technology [1] , [2] . Both logic [3] and storage devices [4] have been proposed based on the controlled propagation of magnetic DWs, achieved through the application of a magnetic field or a current. These two methods, schematically depicted in Fig. 1a,b , share a major disadvantage. For applications, it is necessary to propagate DWs in a controlled manner through a device. Local control of the DWs is therefore required, but none of these methods can be used to accomplish this. 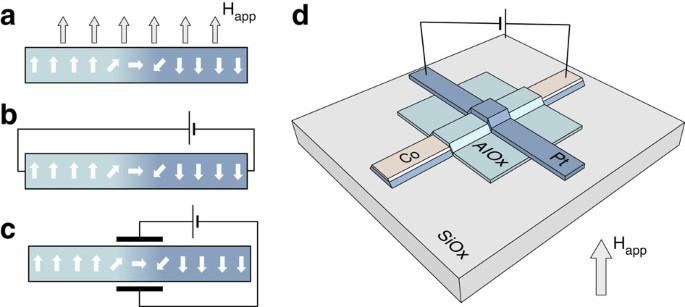Figure 1: Schematic overview of methods to control DW motion. In (a) and (b), the experimentally well-established field- and current-induced DW motion are depicted. In (c), the here-proposed mechanism is shown, namely DW manipulation by an electric field. (d) Overview of the lateral structure of the sample to study DW motion under influence of an electric field. Figure 1: Schematic overview of methods to control DW motion. In ( a ) and ( b ), the experimentally well-established field- and current-induced DW motion are depicted. In ( c ), the here-proposed mechanism is shown, namely DW manipulation by an electric field. ( d ) Overview of the lateral structure of the sample to study DW motion under influence of an electric field. Full size image A new and promising method to control PMA in thin films is the application of an electric field perpendicular to the film plane. This effect has first been demonstrated in semiconducting magnetic materials at cryogenic temperatures [5] , and has more recently been demonstrated at room temperature in ferromagnetic metals [6] , [7] . The prospect of low-power voltage-controlled magnetic switching has recently led to a large number of experimental observations of the effect in various materials [6] , [7] , [8] , [9] , [10] , [11] , [12] , [13] , [14] , [15] , [16] , [17] , demonstrating the manipulation of properties such as magnetic anisotropy [7] , saturation magnetization [12] , and Curie temperature [17] . Theoretical studies into the nature of the electric-field effect suggest that charging of the ferromagnet/oxide interface changes the occupation of surface states, modifying the net anisotropy [18] . Very recently, the first experimental demonstrations of voltage-induced switching have been reported, showing the large potential of voltage controlled spintronics [19] , [20] . Here we explore a novel application of electric field control of magnetism, namely DW motion. Because of the low power costs and compatibility with contemporary technology, controlling DWs with an electric field could be an important addition to the toolbox of future spintronics. The concept of our experiments is schematically depicted in Fig. 1c . By applying an electric field perpendicular to a thin film, we aim to charge the interface and hereby locally change the anisotropy. As DW motion is affected by the anisotropy, we measure the DW velocity modification due to the electric field. Our measurements demonstrate that DW motion in materials with PMA can be significantly increased or decreased by an electric field, and control of DW motion over an order of magnitude is observed. Detailed analysis of the measurements shows that this large control of DW motion can be attributed to a change of PMA in the creep regime. Our observations show that electric field controlled DW motion could be an important tool for the realization of memory and logic devices based on propagation of DWs. Experimental details For the first experiments presented here, Pt/Co/AlOx is used as the magnetic thin film. There are three reasons for choosing this material. First, it shows large PMA at room temperature [21] . Second, the material is extremely interesting for future DW devices, as current-induced DW velocities are reported up to 100 m s −1 (ref. 22 ). Finally, thin AlOx films have proven to be excellent insulators in magnetic tunnel junctions [23] , [24] . A schematic overview of the fabricated samples is shown in Fig. 1d . The bottom electrode consists of a 4 nm platinum layer with a 0.8 nm cobalt layer on top. A sheet of ~3.8 nm AlOx functions as an insulating barrier between the bottom and top electrode, and induces PMA at the Co interface. A 4 nm platinum layer is used as the top electrode. The procedure for sample preparation is described in the Methods section. The junction area is ~220 μm×180 μm and its resistance is three orders of magnitude larger than that of the leads, which means that the junction can be considered an ideal capacitor. The non-ohmic current-voltage characteristic ( Supplementary Fig. S1 ) is another indication of good insulating properties of the barrier. All prepared samples show PMA with 100% remanence. All measurements were performed at room temperature using a Kerr microscope, with which the magnetization reversal can be investigated in real-time. The relatively large size of the junctions allows for accurate optical measurement of DW motion, as it takes relatively long for DWs to propagate through the junction. In experiments, the magnetization is first saturated perpendicular to the plane. At t =0, a magnetic field is instantaneously applied in the opposite direction. Kerr microscopy images are recorded at 16 frames per second. Typical results are depicted in Fig. 2a for an applied magnetic field B of 23 mT and three values of the bias voltage V . In all experiments, DWs nucleate at the edges of the magnetic strip and propagate towards the centre, where they subsequently annihilate. This behaviour results from strongly reduced nucleation fields at the edges of the magnetic strip, caused by small thickness variations due to the contact mask deposition technique. In all experiments, the two nucleated DWs move with approximately the same speed towards the centre of the junction. 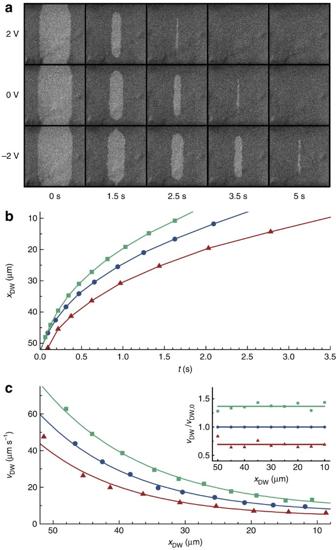Figure 2: Typical measurements of electric-field controlled DW motion. (a) Kerr microscopy images of magnetization reversal in a constant magnetic field of 23 mT. The reversal is followed as a function of time for three values ofV. The visible part of the junction in each image is ~180 μm wide. (b) DW position as a function of time for 2 V (green), 0 V (blue) and −2 V (red) atB=23 mT. The small symbols are measurements, whereas the large ones are averaged data to determinevDWfrom. (c) DW velocity as a function of position atB=23 mT, obtained by differentiating the data in (b). The inset shows the relative change ofvdwas a function ofxDW. Lines are a guide to the eye. Figure 2: Typical measurements of electric-field controlled DW motion. ( a ) Kerr microscopy images of magnetization reversal in a constant magnetic field of 23 mT. The reversal is followed as a function of time for three values of V . The visible part of the junction in each image is ~180 μm wide. ( b ) DW position as a function of time for 2 V (green), 0 V (blue) and −2 V (red) at B =23 mT. The small symbols are measurements, whereas the large ones are averaged data to determine v DW from. ( c ) DW velocity as a function of position at B =23 mT, obtained by differentiating the data in ( b ). The inset shows the relative change of v dw as a function of x DW . Lines are a guide to the eye. Full size image Voltage-dependent DW propagation in Co/AlOx From the Kerr microscopy images, it becomes immediately clear that the DW velocity is sensitive to the bias voltage. For a positive voltage, the DW velocity is increased, whereas a negative voltage decreases the DW velocity. This demonstrates that DWs are not only controllable by a current or an applied field, but also by a bias voltage, which is an important step towards future applications. Although some effect on DW propagation has been indirectly measured in semiconductors at cryogenic temperatures [25] , this is the first direct demonstration of actually controlling DW motion by an electric field in metallic ferromagnets. In Fig. 2b , the DW distance to the centre of the junction, x DW , is plotted as a function of time. The enhancement of the DW velocity near the edge of the sample is a direct result of the deposition profile. The DW velocity v DW is calculated by differentiating x DW with respect to time. The resulting v DW is shown in Fig. 2c as a function of position on the junction. Again, clearly the influence of V on the DW motion can be observed. A positive (negative) voltage is seen to increase (decrease) v DW across the entire sample. Another observation is that v DW converges to some non-zero value for large x DW , indicating that the junction is homogeneous at the centre. The relative change v DW / v DW,0 is plotted as a function of x DW in the inset of Fig. 2c , where v DW,0 is v DW at zero bias. v DW / v DW,0 is observed to be constant over the junction, hence the effect of the electric field on the velocity of the DW is not affected by the deposition profile. We believe that our observations of electric-field control of DW motion are of significant relevance for earlier reports, discussing electric-field-induced coercivity changes [6] , [15] , [16] . In Fig. 3 , hysteresis loops measured with polar MOKE for different bias voltages ( Fig. 3a ) are compared with simulations (Methods) based on magnetization reversal due to DW propagation ( Fig. 3b ). The simulated voltage-induced changes of the coercive field B C are in agreement with the experimentally obtained values. Therefore, we can fully explain changes in the coercivity by the sensitivity of DW motion to the electric field. This means that care should be taken when using the coercive field as a measure for the electric-field-induced changes in PMA. 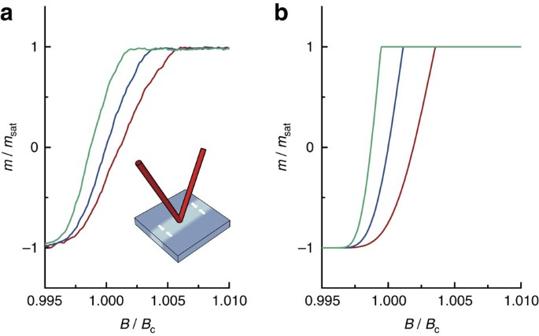Figure 3: Effect of electric-field controlled DW motion on MOKE loops. (a) Normalized polar MOKE measurements on a Co(1.0 nm)/AlOx(3.8 nm) junction for bias voltages of 2.5 V (green), 0 V (blue) and −2.5 V (red). The image shows a schematic overview of the measurement procedure. (b) Simulated MOKE traces for the junction fromFig. 2. The measured change of the coercive fieldBCby a voltage can be fully related to a change in DW creep motion. Figure 3: Effect of electric-field controlled DW motion on MOKE loops. ( a ) Normalized polar MOKE measurements on a Co(1.0 nm)/AlOx(3.8 nm) junction for bias voltages of 2.5 V (green), 0 V (blue) and −2.5 V (red). The image shows a schematic overview of the measurement procedure. ( b ) Simulated MOKE traces for the junction from Fig. 2 . The measured change of the coercive field B C by a voltage can be fully related to a change in DW creep motion. Full size image Electric field control in the creep regime We confirm that the observed control of DW motion is not related to the current ( Supplementary Figs S2 and S3 ; Supplementary Methods ), and must therefore be attributed to electric field-induced modification of material properties. For the small DW velocities observed in the present PMA devices, motion is governed by DW creep [26] , that is, the DW propagates by thermal activation through a disordered potential landscape. In the creep regime, v DW is given by [27] : where U c is an energy constant related to the height of the disorder-induced pinning barrier, and B crit is the field at which the DW pinning energy is equal to the Zeeman energy. Both these parameters depend on the magnetic properties of the sample, which are altered by the electric field. In the Supplementary Methods , we show that the exponent in equation (1) scales approximately linearly with the voltage, assuming that the perpendicular anisotropy scales linearly with voltage, which is supported by Shiota et al . [13] , and pinning is caused by variations in the anisotropy over the sample. The derivation shows that a voltage-induced change in PMA, be it through a change of the surface anisotropy or the saturation magnetization, should be at the origin of the demonstrated sensitivity of v DW to the electric field. To validate whether this creep analysis holds for our samples, the DW velocity at a specific position on the junction ( x DW =20 μm) is plotted as a function of B −1/4 in Fig. 4a and as a function of V in Fig. 4b . The inset of Fig. 4a shows the relative voltage-induced change v DW / v DW,0 as a function of B , demonstrating that the driving field does not have a strong influence on the effect. Although the absolute value of the anisotropy energy E PMA cannot be determined from this data, the relative change can be derived by fitting both the field dependence and the voltage dependence with equation (1). First, v 0 and the typical energy barrier in absence of an electric field are obtained by fitting the magnetic-field dependence from Fig. 4a . Hereafter, the relative change in PMA is obtained by fitting the voltage dependence from Fig. 4b while assuming that the barrier scales linearly with E PMA and V , as derived in the Supplementary Methods . The fits yield a change of 1.9±0.1% nm V −1 , which means that applying 1 V nm −1 alters the PMA by almost 2%. To determine the absolute change in anisotropy, hard-axis MOKE measurements were performed to obtain E PMA , yielding a value of 0.7±0.1 mJ m −2 . The electric-field-induced change in PMA is thus 14±2 fJV −1 m −1 , which is too small to accurately detect in MOKE measurements. However, with this modest change in PMA, we were able to affect v DW by a factor of four by applying just a few volts. 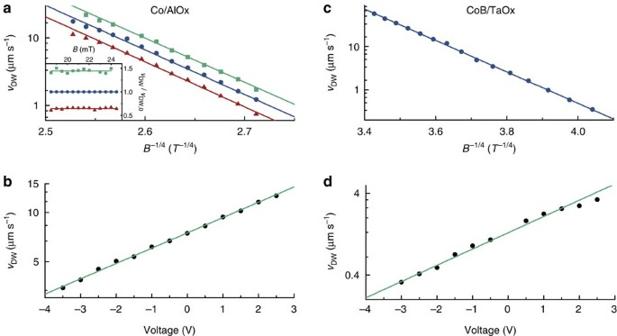Figure 4: DW velocity close to the centre of the junction for a Co/AlOx and CoB/TaOx stack. In (a) and (c),vDWis plotted as a function ofH−1/4for Co/AlOx and CoB/TaOx, respectively. In (a), the measurements are performed for 2 V (green), 0 V (blue) and −2 V (red), whereas, in (c), only the trace at 0 V is depicted. In (b) and (d),vDWis plotted as a function of the applied voltage in an applied field of 22 mT and 5 mT respectively. For CoB/TaOx, control ofvDWis observed over an order of magnitude. The inset of (a) showsvDW/vDW,0as a function of driving field. The lines in all graphs are fits with a creep law allowing for a voltage dependence of the anisotropy. Figure 4: DW velocity close to the centre of the junction for a Co/AlOx and CoB/TaOx stack. In ( a ) and ( c ), v DW is plotted as a function of H −1/4 for Co/AlOx and CoB/TaOx, respectively. In ( a ), the measurements are performed for 2 V (green), 0 V (blue) and −2 V (red), whereas, in ( c ), only the trace at 0 V is depicted. In ( b ) and ( d ), v DW is plotted as a function of the applied voltage in an applied field of 22 mT and 5 mT respectively. For CoB/TaOx, control of v DW is observed over an order of magnitude. The inset of ( a ) shows v DW / v DW,0 as a function of driving field. The lines in all graphs are fits with a creep law allowing for a voltage dependence of the anisotropy. Full size image Increasing the effect by material engineering From the creep law, we expect that v DW is affected by the relative change in PMA rather than an absolute energy change. To increase the influence of the electric field on v DW , junctions identical to Co/AlOx were fabricated, in which only the magnetic and the insulating layer are replaced by different materials. To reduce PMA and increase magnetic field driven DW velocities, we used Co 68 B 32 as the magnetic material [28] . For the barrier, TaOx is used, as the dielectric constant of this material is three times larger than that of AlOx. A larger dielectric constant results in larger charging effects at the interface and subsequently a larger change in PMA. The field and voltage dependences of v DW for a CoB(1 nm)/TaOx(7 nm) junction are depicted in Fig. 4c,d . The field dependence can again be fitted perfectly with the creep law. More importantly, by comparing Fig. 4b,d , it can be concluded that v DW is more sensitive to V in the CoB/TaOx junction compared with the Co/AlOx junction, as the velocity can be changed over an order of magnitude by changing V . The relative change in E PMA is obtained by fitting the data with equation (1), giving 10±0.5% nm V −1 . This corresponds to an absolute change of 28±4 fJV −1 m −1 . Although it is difficult at this point to attribute the larger control of DW motion in CoB/TaOx compared with Co/AlOx to a single changed material property, it demonstrates that, by material engineering, the effect can be significantly increased. Comparing the measured absolute change in E PMA to earlier reports, we see that our values are comparable to measurements in Au/FeCo/MgO (ref. 14 ). However, one can also compare the result to theoretical calculations [13] , [18] , where values are reported ranging from 100 to 200 fJV −1 m −1 . If these values could be obtained in real devices, we can extrapolate from our measurements a voltage-controlled change in DW motion over five orders of magnitude. With such modifications, DWs can be effectively pinned or depinned by the electric field, opening up unique opportunities to control DWs in experiments and devices. To achieve this in an experiment, more research is required to gain precise control of the magnetic properties and the quality of the films, which does not lie within the scope of the present work. Many new devices can be imagined based on controlling DWs with an electric field. An example of such an application is depicted in Fig. 5 . In the racetrack memory proposed by Parkin et al . [4] , which is a shift register based on DW motion, DWs have to be moved in discrete steps, which is suggested to be accomplished by locally pinning the DWs. Pinning by device geometry [29] or ion irradiation [30] has shown to be viable; however, this effect is permanent. The advantage of using an electric field to pin a DW is that the pinning potential can be changed by varying the applied voltage. In the device depicted in Fig. 5 , the DW is depinned from its current location by a positive voltage, whereas a negative voltage pins the DW at its new location. In this manner there is no potential barrier that has to be overcome to depin the DW, significantly lowering the probability of DW overshoot or that a DW will not move at all. We emphasize that by tuning material parameters it should be possible to switch between the flow and creep regime. 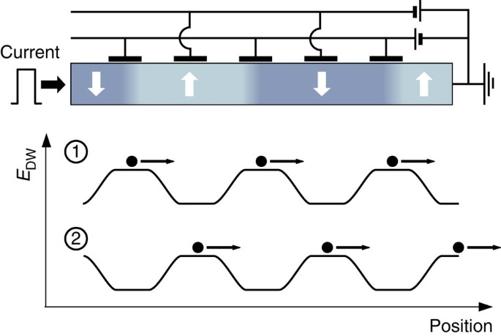Figure 5: Example of an application for electrical control of DW motion in a shift register. Current pulses propagate DWs by spin-transfer torque. Two arrays of electrical gates are positioned on the magnetic wire. By using opposite polarities for the voltages over the two arrays during the current pulse (1), the electric field assists depinning at the starting location and pins the DW at the final location. At the next current pulse (2), the polarities are switched, moving the DWs controllably through the magnetic wire. Figure 5: Example of an application for electrical control of DW motion in a shift register. Current pulses propagate DWs by spin-transfer torque. Two arrays of electrical gates are positioned on the magnetic wire. By using opposite polarities for the voltages over the two arrays during the current pulse (1), the electric field assists depinning at the starting location and pins the DW at the final location. At the next current pulse (2), the polarities are switched, moving the DWs controllably through the magnetic wire. Full size image The proposed device is just one of many possible applications of E-controlled DW motion. One major advantage of the approach is that it can be readily integrated in existing technology. Furthermore, the technique is compatible with various new spintronic devices based on DW motion. Finally, the intrinsic low power consumption of controlling magnetism with an electric field [31] enlarges its potential. We envision that the measurements presented here will trigger efforts to both increase the magnitude of the effect and to develop new applications, providing an important first step towards a new type of low power room temperature magnetic devices, in which DWs can be locally controlled in real-time by a voltage. Sample preparation Samples were grown by DC sputtering and structured using a contact mask technique. A Pt(4 nm)/Co(0.8 nm) or Pt(4 nm)/CoB(0.8 nm) bottom electrode is deposited on a Si(B)/SiOx substrate. The wire is covered by two Al(1.5 nm) or Ta(1.4 nm) sheets, which are both plasma oxidized for 10 minutes at a pressure of 0.1 mbar and a power of 30 W, ensuring both insulating properties of the barrier and PMA of the magnetic film. Using two sheets instead of one reduces the chance of pinholes and increases the breakdown voltage. The nominal thickness of the two layers after plasma oxidation is ~3.8 nm and ~7.0 nm for the AlOx and TaOx, respectively. Finally, a Pt(4 nm) crossbar electrode is sputtered on top. MOKE loop simulations Polar MOKE traces for different bias voltages are simulated for a sample with identical magnetic properties as the junction in Fig. 4a,b . The perpendicular magnetization of the sample M z is assumed to depend solely on the DW position x , where − w /2≤ x ≤ w /2 with w =220 μm, hence reversal of the junction is simplified to a one-dimensional problem. DWs appear as step functions propagating from either side of the junction towards the centre. For each time step, the velocity v ( x , B , V ) is given by the DW creep law, using parameter values derived directly from experiments in Fig. 4a,b . The resulting MOKE signal is simulated by multiplying M z ( x ) with a Gaussian laser spot centred at x =0 with a FWHM of 15 μm. How to cite this article: Schellekens, A. J. et al . Electric-field control of domain wall motion in perpendicularly magnetized materials. Nat. Commun. 3:847 doi: 10.1038/ncomms1848 (2012).